Multiple exposures to drought 'train' transcriptional responses inArabidopsis Pre-exposure to stress may alter plants' subsequent responses by producing faster and/or stronger reactions implying that plants exercise a form of 'stress memory'. The mechanisms of plants' stress memory responses are poorly understood leaving this fundamental biological question unanswered. Here we show that during recurring dehydration stresses Arabidopsis plants display transcriptional stress memory demonstrated by an increase in the rate of transcription and elevated transcript levels of a subset of the stress–response genes (trainable genes). During recovery (watered) states, trainable genes produce transcripts at basal (preinduced) levels, but remain associated with atypically high H3K4me3 and Ser5P polymerase II levels, indicating that RNA polymerase II is stalled. This is the first example of a stalled RNA polymerase II and its involvement in transcriptional memory in plants. These newly discovered phenomena might be a general feature of plant stress–response systems and could lead to novel approaches for increasing the flexibility of a plant's ability to respond to the environment. Plants' responses to abiotic stresses involve coordinated actions to change cellular physiology and gene expression patterns [1] . A previous exposure to a stress may alter a plant's subsequent stress response by producing faster and/or stronger reactions that may provide the benefits of enhanced protection [2] , [3] . Altered responses to consecutive stresses imply that plants exercise a form of 'stress memory' [4] . For example, tobacco plants pre-exposed to methyl jasmonate increased nicotine pools 2 days earlier when exposed again as compared with plants without previous exposure [5] ; Pretreatment of plants with salicylic acid or its synthetic analogue, benzothiadiazole S -methylester, resulted in increased transcription from a subset of genes upon a subsequent stress [6] , [7] . Some stress memory effects could be perpetuated to the next generation, as observed with flagellin or ultraviolet radiation [8] treatments. The molecular mechanisms associated with stress memory are largely unknown. Accumulation of dormant signalling molecules that are recruited only on exposure to stress, or proteins involved in their synthesis, have been proposed [2] . Epigenetic control systems offer an alternative mechanism for responses that are dynamic and persistent: a gene, or a network, is activated in response to a stimulus, but once the stimulus is removed, a mark could be left to facilitate altered, quicker or more potent responses to subsequent stresses. Therefore, epigenetic systems may act as the conduit for environmental cues initiating both short- and long-term changes in gene expression in response to a stress. The formal definition of epigenetics includes a heritable (mitotic or meiotic) component. However, the finding that the functional states of neurons, which almost never divide, involve epigenetic phenomena [9] has prompted a refined definition suggesting a broader meaning that excludes the strict requirement for heritability [10] . In this paper, we use the term 'epigenetics' within this broader context as we study responses in leaf cells that have predominantly ceased division. It is important to emphasize also that we distinguish between a chromatin mark (reflecting a modification that is dynamically associated with a process, but is removed at the conclusion of that process) and an epigenetic mark to imply persistence longer than the initial stimulus that caused the chromatin mark and that affects subsequent performances of the gene. We define 'transcriptional memory' to mean that a type of information persists after the plant has recovered from the initial stress and that the 'memory' influences subsequent transcriptional responses. We found that during recurring dehydration stresses Arabidopsis plants demonstrate transcriptional memory of the stress as displayed by increased rates of transcription and elevated transcript levels from a subset of the stress–response genes (trainable genes). The transcriptional memory is associated with two distinct marks found only at the trainable genes during their recovery from stress-induced transcription: high levels of trimethylated histone H3 Lys4 (H3K4me3) nucleosomes and stalled Ser5P Pol II. In contrast, H3K4me3 and Ser5P dynamically increase when non-trainable genes are induced and then decrease to basal levels during the recovery. At the trainable genes, H3K4me3 and Ser5P polymerase II (Pol II) persist as 'memory marks' for as long as the transcriptional memory responses last. The low transcription rates and high Ser5P Pol II levels during the watered recovery conditions provide the first evidence of a stalled RNA Pol II in plants. Dehydration stress-trained Arabidopsis plants To determine whether plants retain a memory of a previous dehydration stress (trained plants), we developed a repetitive dehydration/rehydration system of air-drying for 2 h and rehydration for 22 h (Methods). Non-trained plants wilted faster than trained plants ( Fig. 1a ) and their leaves lost water at a faster rate than trained plants ( Fig. 1b ). The leaf relative water content (RWC) at the beginning of each stress treatment (measured at the end of the R1–R3 recovery periods) was similar to the RWC of initial preinduced watered (W) state ( Fig. 1c ). The results showed that despite losing water during air exposure, rehydration brought the RWC to the initial prestress levels, indicating plants have fully recovered and start each dehydration stress test at similar initial RWCs. These results are consistent with drought hardening observed in horticultural plants [11] , supporting the idea that trained plants alter their responses after an initial dehydration stress. 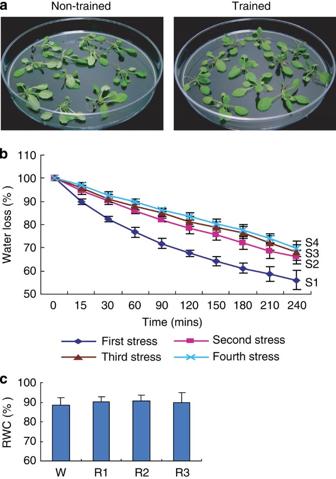Figure 1: Response to dehydration stress of trained or non-trained plants. (a) Appearance of 3-week-oldArabidopsisplants to 1-h exposure to air if not previously stressed (non-trained) or previously stressed with three consecutive cycles of stress/recovery treatments (trained). (b) Fresh weights of leaves, after air drying for the indicated times, for plants experiencing their first stress (dark blue line) or for trained plants exposed to a second (red line), third (brown line) or fourth (light blue line) stress cycles. Experiments inawere repeated at least 5 times. Three independent experiments were performed forb, each with three replicates, each containing 8–10 leaves. The representative experiment shown indicates the mean±s.e.m.,n=3 replicates. (c) Relative water content (RWC) measured during the initial watered (W) state and on recovery (R1–R3) from one or more stresses, before a subsequent dehydration stress (second, third or fourth stress) as described inb. Figure 1: Response to dehydration stress of trained or non-trained plants. ( a ) Appearance of 3-week-old Arabidopsis plants to 1-h exposure to air if not previously stressed (non-trained) or previously stressed with three consecutive cycles of stress/recovery treatments (trained). ( b ) Fresh weights of leaves, after air drying for the indicated times, for plants experiencing their first stress (dark blue line) or for trained plants exposed to a second (red line), third (brown line) or fourth (light blue line) stress cycles. Experiments in a were repeated at least 5 times. Three independent experiments were performed for b , each with three replicates, each containing 8–10 leaves. The representative experiment shown indicates the mean±s.e.m., n =3 replicates. ( c ) Relative water content (RWC) measured during the initial watered (W) state and on recovery (R1–R3) from one or more stresses, before a subsequent dehydration stress (second, third or fourth stress) as described in b . Full size image Trainable and non-trainable Arabidopsis genes Trained plants also responded differently at the transcriptional level. We analysed four genes widely used as markers for dehydration-inducible genes ( RD29A, RD29B, RAB18 and COR15A (refs 12 , 13 , 14 , 15 )) and observed two distinct types of expression patterns during repeated stresses ( Fig. 2a,b ). The RD29A and COR15A genes repetitiously increased their transcripts to about the same level during each stress (non-trainable genes). In contrast, RD29B and RAB18 produced considerably higher transcript levels during one or more subsequent stresses relative to the initial stress (the trainable genes). A critical result is that during the recovery (watered) states both the non-trainable and the trainable genes return to their initial (non-stressed) transcript levels. Restoration of each gene's activity to its prestressed level when stress signalling was alleviated indicates lack of a persistent induction. Return to baseline transcript levels from the trainable genes during recovery, together with a higher induction level on a following stress, illustrates the concept of 'transcriptional memory'. 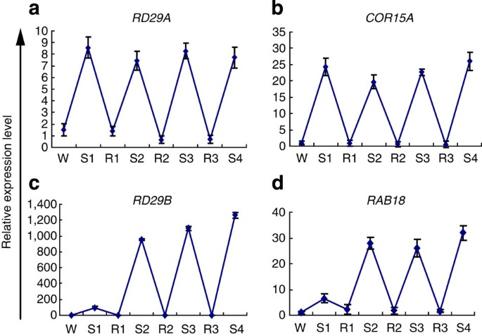Figure 2: Transcript levels of non-trainable and trainable genes in plants before and after single or multiple dehydration stresses. RNA was isolated from watered plants (initial state defined as watered, W) and from plants subjected to one to four dehydration stresses of 2 h of air drying (S1–S4) separated by 22-h intervals of watered recovery treatments (R1–R3). Transcript levels for (a)RD29A; (b)COR15A; (c)RD29B; (d)RAB18genes were measured by reverse transcription and real-time quantitative PCR.UBQ10was used as an internal control. Genes are considered trained if the transcript level in S1 is considerably less than in subsequent stresses, as occurring forRD29BandRAB18.Experiments were repeated at least three times, each with three replicates, and the representative experiment shown indicates the mean±s.e.m.,n=3 replicates. Figure 2: Transcript levels of non-trainable and trainable genes in plants before and after single or multiple dehydration stresses. RNA was isolated from watered plants (initial state defined as watered, W) and from plants subjected to one to four dehydration stresses of 2 h of air drying (S1–S4) separated by 22-h intervals of watered recovery treatments (R1–R3). Transcript levels for ( a ) RD29A ; ( b ) COR15A ; ( c ) RD29B ; ( d ) RAB18 genes were measured by reverse transcription and real-time quantitative PCR. UBQ10 was used as an internal control. Genes are considered trained if the transcript level in S1 is considerably less than in subsequent stresses, as occurring for RD29B and RAB18. Experiments were repeated at least three times, each with three replicates, and the representative experiment shown indicates the mean±s.e.m., n =3 replicates. Full size image To establish whether transcriptional memory was carried also by other dehydration stress–response genes, we searched for genes displaying increased transcript levels in multiply stressed plants. Five additional non-trainable genes ( Supplementary Fig. S1a,b ) and five additional trainable genes were identified ( Supplementary Fig. S1a,c ). Collectively, our results uncovered a hitherto unknown existence of two distinct subsets within the dehydration stress–response gene fraction: the repetitively responding non-trainable genes and the trainable genes, which increased the magnitude of their subsequent transcriptional response, relative to their initial stress response. Transcription rates of trainable and non-trainable genes Restoration of transcript levels to the basal non-induced levels during the watered recoveries indicated that response genes' mRNAs were not persisting from one stress to the next. Whether elevated transcript levels were due to increased rates of transcription was determined by nuclear run on assays. The non-trainable RD29A and COR15A genes had similar transcription rates during each stress treatment ( Fig. 3a,b ). In contrast, the trainable RD29B and RAB18 genes displayed threefold higher transcription rates during the repeated stress (S4) relative to their rates during the first (S1) stress ( Fig. 3c,d ). Similar transcription rates during the initial (prestressed) and the recovery (watered) phases for both the trainable and non-trainable genes indicated that in the absence of dehydration stress, transcription was restored to the initial levels and that the increased transcript production by the trainable genes was regulated, at least in part, at the level of transcription. 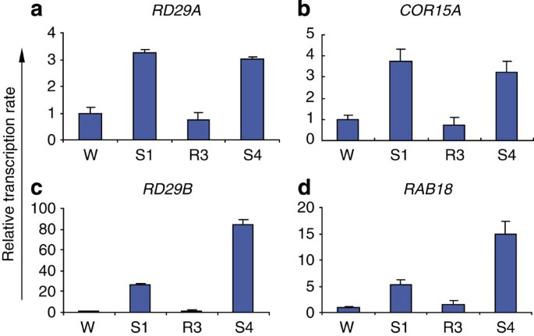Figure 3: Nuclear run on assays of non-trained or trained plants. Nuclei were isolated from non-stressed watered (W), singly (S1) or repetitively stressed plants. The repetitively stressed plants were dehydration stressed 3 times and then nuclei isolated before (recovery R3) or during a fourth dehydration stress (S4). Isolated nuclei were used in run on transcription reactions containing biotin-UTP to label newly synthesized transcripts. The nascent biotin-labelled transcripts were purified by binding to streptavidin beads and quantitated by quantitative PCR (qPCR) for (a)RD29A; (b)COR15A; (c)RD29B; (d)RAB18genes. Labelling experiments were repeated at three times, each with three reverse transcription–qPCR measurements, and the representative experiment shown indicates the mean+s.e.m.,n=3 replicates.UBQ10was used as internal control. Figure 3: Nuclear run on assays of non-trained or trained plants. Nuclei were isolated from non-stressed watered (W), singly (S1) or repetitively stressed plants. The repetitively stressed plants were dehydration stressed 3 times and then nuclei isolated before (recovery R3) or during a fourth dehydration stress (S4). Isolated nuclei were used in run on transcription reactions containing biotin-UTP to label newly synthesized transcripts. The nascent biotin-labelled transcripts were purified by binding to streptavidin beads and quantitated by quantitative PCR (qPCR) for ( a ) RD29A ; ( b ) COR15A ; ( c ) RD29B ; ( d ) RAB18 genes. Labelling experiments were repeated at three times, each with three reverse transcription–qPCR measurements, and the representative experiment shown indicates the mean+s.e.m., n =3 replicates. UBQ10 was used as internal control. Full size image Distribution of the elongating (Ser2P) Pol II Next we investigated the possible roles of RNA Pol II and the chromatin histone H3K4me3 modification in the different transcriptional behaviour of the trainable and the non-trainable genes. The distribution of the actively elongating form of Pol II, phosphorylated at serine 2 (Ser2P) of the consensus (Y 1 S 2 P 3 T 4 S 5 P 6 S 7 ) 34 CTD repeat, was analysed during the induced and recovery phases of the dehydration-stress cycle. Active transcription elongation is associated with high Ser2P levels accumulating towards the 3′-ends of actively transcribed genes [16] . In agreement, the Ser2P distribution profiles showed a peak towards the 3′-ends of both the non-trainable and the trainable genes when induced by stress ( Fig. 4a,b ). 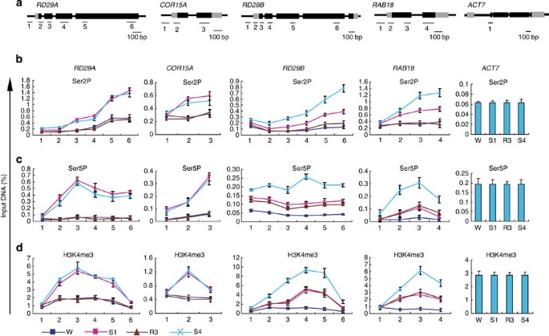Figure 4: Profiles of Pol II and of H3K4me3 at the non-trainable and trainable genes. (a) Schematic diagram of the genes, with the promoter region (to left), the 5′ untranslated region (grey box), exons (dark box), introns (thin lines between exons) and indicating the regions (1 to 6) analysed by chromatin immunoprecipitation and real-time qPCR (ChIP–qPCR). (b–d)ChIP–qPCR analysis of the amounts of specific modifications present at regions 1–6 for the non-stressed watered (W, dark blue), singly stressed (S1, red) and trained plants (three stress cycles) before recovery (R3, brown) or during a fourth dehydration stress (S4, light blue). The results withACT7are shown as an internal control; (b) distribution profiles of Ser2P Pol II; (c) distribution profiles of Ser5P Pol II; (d) distribution profiles of H3K4me3. Experiments were repeated at least four times, each with three replicates, and the representative experiment shown indicates the mean±s.e.m.,n=3 replicates. Figure 4: Profiles of Pol II and of H3K4me3 at the non-trainable and trainable genes. ( a ) Schematic diagram of the genes, with the promoter region (to left), the 5′ untranslated region (grey box), exons (dark box), introns (thin lines between exons) and indicating the regions (1 to 6) analysed by chromatin immunoprecipitation and real-time qPCR (ChIP–qPCR). ( b – d) ChIP–qPCR analysis of the amounts of specific modifications present at regions 1–6 for the non-stressed watered (W, dark blue), singly stressed (S1, red) and trained plants (three stress cycles) before recovery (R3, brown) or during a fourth dehydration stress (S4, light blue). The results with ACT7 are shown as an internal control; ( b ) distribution profiles of Ser2P Pol II; ( c ) distribution profiles of Ser5P Pol II; ( d ) distribution profiles of H3K4me3. Experiments were repeated at least four times, each with three replicates, and the representative experiment shown indicates the mean±s.e.m., n =3 replicates. Full size image The Ser2P distribution during both the non-induced and the stress-induced phases of the cycle provided independent support that the transcript levels measured in recovery or during stress were regulated at the level of transcription. First, transcription of both trainable and non-trainable genes during watered recovery returns to their initial levels in watered plants, as Ser2P levels during R3 are similar to those in watered. Second, during stress-induced transcription, the trainable ( RD29B and RAB18 ) genes accumulate higher Ser2P in S4 than in S1, consistent with their enhanced transcription. Contrasting this pattern, the non-trainable ( RD29A and COR15A ) genes accumulate similar Ser2P amounts during S1 or S4, consistent with their transcriptional responses. The distribution profiles for the elongating Ser2P were also established for the additional five non-trainable and five trainable genes ( Supplementary Fig. S1a–c ). The results from these non-trainable and trainable groups were similar to the patterns displayed by the non-trainable RD29A and COR15A , and trainable RD29B and RAB18 , respectively. Thereby, Ser2P levels correlated with transcription rates and transcript levels. As the operational definition of memory marks is that they must last longer than the stimulus, we conclude that Ser2P does not function as a memory mark. Stalled Pol II and H3K4me3 as memory marks The distribution of the phosphorylated serine 5 form of Pol II (Ser5P), associated with transcription initiation/early elongation or pausing/stalling [16] , [17] , was analysed next. Ser5P levels follow the transcription rates and transcript abundances from the non-trainable RD29A and COR15A genes during all treatments: the initial (S1) and repetitively stressed states (S4) show similar Ser5P levels; similar levels were also found in the prestressed (W) and recovery (R3) states ( Fig. 4c ). These patterns were confirmed in the five additional non-trainable genes as well ( Supplementary Fig. S1b ). For the trainable genes, the Ser5P patterns were different: higher for the repetitively stressed (S4) than for singly stressed (S1) plants ( Fig. 4c , Supplementary Fig. S1c ), consistent with their transcript levels ( Fig. 2 ) and transcription rates ( Fig. 3 ). The most remarkable difference, however, was the atypically high Ser5P level in the watered conditions, despite the low transcription of RD29B and RAB18 . During recovery (R3), Ser5P was retained at levels similar to the levels generated during the first stress (S1) at RD29B and RAB18 ( Fig. 4c ). Elevated Ser5P was also displayed by the five additional trainable genes during recovery ( Supplementary Fig. S1c ). Retention of high Ser5P presence at trained genes during the watered recovery when transcription rates were low suggested that Ser5P Pol II was stalled. Stalled Pol II was found only at the trainable dehydration stress–response genes during their recovery from an induced transcription. Thereby, elevated Ser5P Pol II during recovery behaves as a memory mark from a previously active state. To determine whether transcriptional memory was also associated with a histone modification, we analysed the H3K4me3 profiles. For all non-trainable genes, the H3K4me3 modification increased to similar levels on each stress induction and decreased to baseline levels in watered plants ( Fig. 4d and Supplementary Fig. S1b ). For the trainable genes, H3K4me3 also increased on gene induction, but repetitively stressed (S4) plants displayed higher H3K4me3 than singly stressed (S1) plants ( Fig. 4d ; Supplementary Fig. S1c ). This pattern is in agreement with their increased transcript abundances and transcription rates ( Figs 2b,c, and 3b,c ). Importantly, however, during recovery (R3) the trainable genes in repetitively stressed plants had higher H3K4me3 levels than in the non-stressed state (F); the elevated H3K4me3 levels were similar to those of the singly stressed (S1) plants ( Fig. 4d ), indicating that H3K4me3 modification was retained on the nucleosomes of the trainable genes during the recovery states. Retention of high H3K4me3 levels in R3, comparable with S1 was also displayed by the other five trainable genes analysed ( Supplementary Fig. S1c ). Furthermore, analyses of histone H3 distribution at representative trainable, or non-trainable, genes revealed similar nucleosome levels during the prestressed (W) and the last recovery (R3) states ( Fig. 5 ). The higher H3K4me3 levels in R3 relative to those in watered, thereby, reflect H3K4me3 modifications retained from the preceding transcription. 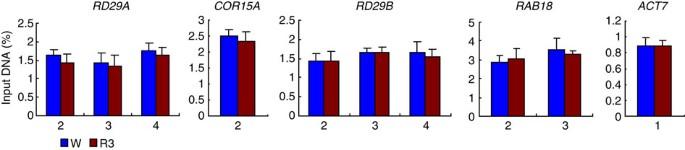Figure 5: Nucleosomal distribution at the non-trainable and trainable genes. The columns represent the amounts of Histone H3 measured by ChIP–PCR with antibodies specific for histone H3. Numbers under the columns indicate tested regions along the gene sequences as indicated inFig. 4a. Data from fresh non-stressed tissues (blue columns) and stressed plants in the R3 recovery interval (brown columns) are shown for the non-trainableRD29A,COR15Aand the trainableRD29B,RAB18genes. Data are from three biological sample replicas. Figure 5: Nucleosomal distribution at the non-trainable and trainable genes. The columns represent the amounts of Histone H3 measured by ChIP–PCR with antibodies specific for histone H3. Numbers under the columns indicate tested regions along the gene sequences as indicated in Fig. 4a . Data from fresh non-stressed tissues (blue columns) and stressed plants in the R3 recovery interval (brown columns) are shown for the non-trainable RD29A , COR15A and the trainable RD29B , RAB18 genes. Data are from three biological sample replicas. Full size image Therefore, at the non-trainable genes, H3K4me3 acts as a reversible chromatin mark dynamically changing with transcript levels. At the trainable genes, H3K4me3 acts as a persistent epigenetic mark associated with the transcriptional memory displayed by these genes. Length of the transcriptional memory persistence To establish how long transcriptional memory can persist in the absence of inducing signals, trained and untrained plants were watered for 3, 5 or 7 days in soil, and then their transcript levels were measured before and after a subsequent dehydration stress. In trained plants, after 3 or 5 days of recovery, the RD29B and RAB18 genes displayed super-induced transcript levels when exposed to dehydration stress. After 7 days, however, when plants were stressed, the RD29B and RAB18 transcripts were induced at non-trained levels ( Fig. 6a,b ). The non-trainable ( RD29A and COR15A ) genes showed little variation in their responses on any of these days ( Fig. 6c,d ). We conclude that dehydration stress-induced transcriptional memory persists for 5 days, but is lost after 7 days, under watered conditions. 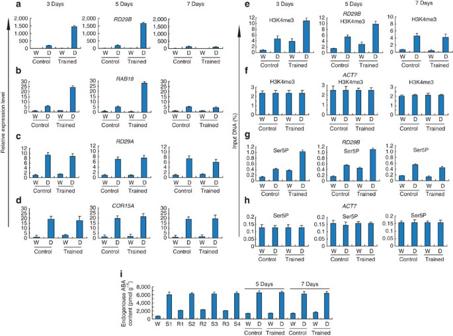Figure 6: Length of the transcriptional memory in trained plants. The relative levels of mRNA of trained plants after a recovery period under watered conditions for 3 or more days, before and after a subsequent dehydration stress are shown ina–d. Plants were not stressed (Control) or were dehydration stressed 4 times (Trained), with 22-h recovery periods before receiving water in soil for 3, 5 or 7 days (first, second and third columns, respectively). After the indicated days of watering, plants received water (W) or were dehydration stressed (D) for 2 h before the indicated analyses. (a,b)Transcript levels of the trainable (RD29BandRAB18) genes. (c,d) Transcript levels of the non-trainable (RD29Aand COR15A) genes measured by reverse transcription–quantitative PCR (qPCR).UBQ10was used as an internal control. (e) H3K4me3 levels at theRD29Bgene measured by ChIP–qPCR, relative to ACT7, shown infat the regions showing the peak accumulation of the respective marks at each gene (seeFig. 4for location of the peak regions). (g) Ser5P levels at theRD29Bgene measured by ChIP–qPCR, relative to ACT7 shown inh, at the regions showing the peak accumulation of the respective marks at each gene (seeFig. 4for location of the peak regions). Results from measurements during days 3, 5 or 7 after recovery in soil are shown in the first, second and third columns, respectively. (i) ABA levels before stress (W), after one to four stresses (S1–S4) or one to three recoveries (R1–R3) and before (W) or after a dehydration stress (D) that was initiated after 5 or 7 days of watering of control or trained plants. Experiments ina–cwere repeated at least three times, each with three replicates, and the representative experiments shown indicates the mean+s.e.m.,n=3 replicates. Experiments indwere performed twice, with two replicates, and the representative experiment shown indicates the mean+range,n=2 replicates. Figure 6: Length of the transcriptional memory in trained plants. The relative levels of mRNA of trained plants after a recovery period under watered conditions for 3 or more days, before and after a subsequent dehydration stress are shown in a – d . Plants were not stressed (Control) or were dehydration stressed 4 times (Trained), with 22-h recovery periods before receiving water in soil for 3, 5 or 7 days (first, second and third columns, respectively). After the indicated days of watering, plants received water (W) or were dehydration stressed (D) for 2 h before the indicated analyses. ( a , b) Transcript levels of the trainable ( RD29B and RAB18 ) genes. ( c , d ) Transcript levels of the non-trainable ( RD29A and COR15A) genes measured by reverse transcription–quantitative PCR (qPCR). UBQ10 was used as an internal control. ( e ) H3K4me3 levels at the RD29B gene measured by ChIP–qPCR, relative to ACT7, shown in f at the regions showing the peak accumulation of the respective marks at each gene (see Fig. 4 for location of the peak regions). ( g ) Ser5P levels at the RD29B gene measured by ChIP–qPCR, relative to ACT7 shown in h , at the regions showing the peak accumulation of the respective marks at each gene (see Fig. 4 for location of the peak regions). Results from measurements during days 3, 5 or 7 after recovery in soil are shown in the first, second and third columns, respectively. ( i ) ABA levels before stress (W), after one to four stresses (S1–S4) or one to three recoveries (R1–R3) and before (W) or after a dehydration stress (D) that was initiated after 5 or 7 days of watering of control or trained plants. Experiments in a – c were repeated at least three times, each with three replicates, and the representative experiments shown indicates the mean+s.e.m., n =3 replicates. Experiments in d were performed twice, with two replicates, and the representative experiment shown indicates the mean+range, n =2 replicates. Full size image Next, we analysed how long the memory marks persisted in the absence of induced transcription. We found that at the trainable genes, the high Ser5P Pol II and H3K4me3 levels were also retained for 3 and 5 days, but not for 7 days ( Fig. 6e–h ). Thereby, the similar duration of transcriptional memory and of elevated Ser5P Pol II and H3K4me3 levels strengthens their association and our conclusion that Ser-5P Poll II and H3K4me3 levels function as memory marks at the genes displaying transcriptional memory. Abscisic acid and transcriptional memory The phytohormone ABA induces transcription from Arabidopsis dehydration stress–response genes [15] and was examined as a potential factor in stress memory responses. Endogenous ABA levels repetitiously increased upon each dehydration stress, but returned to low levels during each recovery treatment ( Fig. 6i ). This pattern also occurred after the extended recovery periods, as similar levels of endogenous ABA were produced when plants were stressed after 3, 5 or 7 days recovery in watered soil ( Fig. 6i ). The high ABA levels were similar in each stress cycle and rule out a model wherein higher levels of ABA in subsequent stresses were responsible for the super-induced transcript levels of the trainable genes. The residual amount of ABA after dehydration stress is slightly higher than the initial level in non-stressed plants but, apparently, insufficient to induce transcription in R1–R3. Further, this residual ABA level is present after 3, 5 and 7 days of watering ( Fig. 6i ), even though transcriptional memory is lost after 7 days of watering ( Fig. 6a,b ). The results indicate that induced ABA levels were not sufficient to cause super-induced transcript levels and residual ABA levels were not sufficient to maintain a memory response. Role of ABA-regulated ABRE-binding transcription factors Recent studies have identified ABA-responsive elements (ABREs) AREB1, AREB2 and ARF3 as basic domain leucine zipper transcription factors (TFs) that act as master regulators to cooperatively regulate gene expression from a large number of plant dehydration stress–response genes [18] . These TFs bind to ABREs found in the promoters of ABA-inducible genes and require ABA for their activity. AREB1, AREB2 and ARF3 have largely overlapping functions, therefore we used a plant genotype with mutations in all three genes ( areb1/areb2/abf3 triple mutant) [18] to assess the potential effect of the three TFs on the transcriptional memory response. This analysis revealed that transcript levels from both the non-trainable ( RD29A and COR15A ) and trainable ( RD29B and RAB18 ) genes were strongly diminished in the triple mutant plants ( Fig. 7a–d ). However, despite the strong reduction in transcription, both RD29B and RAB18 produced much higher levels of transcripts in S4 than in S1 ( Fig. 7c,d ), indicating that transcriptional memory was still functional. Thereby, although critical for inducing maximal transcription in response to dehydration stress, AREB1, AREB2 and ARF3 are not essential for the transcriptional memory response. 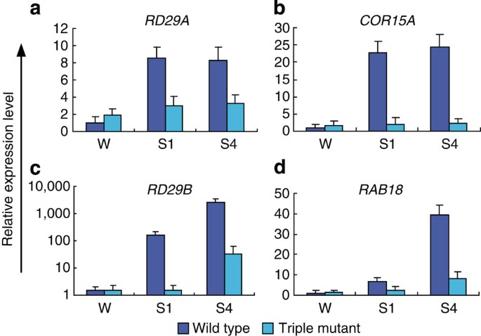Figure 7: The role of three ABA-dependent transcription factors in the transcriptional memory. The effects of three ABA-dependent transcription factors, AREB1, AREB2 and ABF3, were examined in the wild-type (dark blue columns) andareb1/areb2/abf3triple mutant backgrounds (light blue columns) before and after multiple dehydration stresses. Transcript levels were determined in plants during their prestressed (W), first stressed (S1) and fourth stressed (S4) periods. Transcript levels of the non-trainable (a)RD29Aand (b)COR15Agenes. Transcript levels of the trainable (c)RD29Band (d)RAB18genes. Note the scale forRD29Bis logarithmic.UBQ10was used as an internal control. Experiments were repeated two times, each with three replicates, and the representative experiment shown indicates the mean±s.e.m.,n=3 replicates. Figure 7: The role of three ABA-dependent transcription factors in the transcriptional memory. The effects of three ABA-dependent transcription factors, AREB1, AREB2 and ABF3, were examined in the wild-type (dark blue columns) and areb1/areb2/abf3 triple mutant backgrounds (light blue columns) before and after multiple dehydration stresses. Transcript levels were determined in plants during their prestressed (W), first stressed (S1) and fourth stressed (S4) periods. Transcript levels of the non-trainable ( a ) RD29A and ( b ) COR15A genes. Transcript levels of the trainable ( c ) RD29B and ( d ) RAB18 genes. Note the scale for RD29B is logarithmic. UBQ10 was used as an internal control. Experiments were repeated two times, each with three replicates, and the representative experiment shown indicates the mean±s.e.m., n =3 replicates. Full size image Role of ATX1 in transcriptional memory As Arabidopsis Trithorax-like 1 (ATX1) regulates a large number of dehydration stress–response genes [19] , [20] , [21] , its potential role in the memory responses was investigated here. Dehydration-induced transcript levels were strongly diminished in atx1 plants, consistent with its activating role at these genes ( Fig. 8a–d ). However, the trainable RD29B and RAB18 genes still produced increased transcripts in trained, relative to untrained, atx1 plants ( Fig. 8c,d ) and retained H3K4me3 levels at elevated levels during the watered recovery states ( Fig. 8e ). Trained or untrained atx1 plants also showed differences in the rates of leaf water loss, albeit smaller than the differences between trained and untrained wild-type plants ( Fig. 8f ). Together these results indicate that transcriptional memory responses were attenuated in atx1 mutants but stress memory was still occurring. 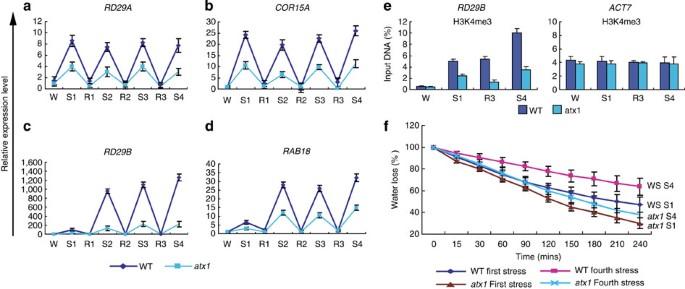Figure 8: Role of ATX1 in the dehydration stress memory. Transcript levels in wild-type (WS, shown in dark blue) oratx1(shown in light blue) plants measured before stress (W), after one to four stresses (S1–S4), or one to three recoveries (R1–R3). Results relative to UBQ10 are shown for the non-trainable (a)RD29A, (b)COR15Aand the trainable (c)RD29Band (d)RAB18genes; (e) H3K4me3 levels measured by ChIP–quatitative PCR during the watered or dehydration stress treatments for WS (dark blue) andatx1(light blue) plants for the trainableRD29Bgene; the profiles of the controlACT7gene is shown in the panel to the right. (f) Rates of water loss from detached leaves of wild-type (WS) oratx1plants during a first or fourth dehydration stresses: dark blue and red lines illustrate data for WS, first and fourth stresses, respectively; brown and light blue lines illustrate data foratx1during the first and fourth stresses, respectively. Experiments were repeated at least twice, each with three replicates, and the representative experiment shown indicates the mean±s.e.m.,n=3 replicates. Figure 8: Role of ATX1 in the dehydration stress memory. Transcript levels in wild-type (WS, shown in dark blue) or atx1 (shown in light blue) plants measured before stress (W), after one to four stresses (S1–S4), or one to three recoveries (R1–R3). Results relative to UBQ10 are shown for the non-trainable ( a ) RD29A , ( b ) COR15A and the trainable ( c ) RD29B and ( d ) RAB18 genes; ( e ) H3K4me3 levels measured by ChIP–quatitative PCR during the watered or dehydration stress treatments for WS (dark blue) and atx1 (light blue) plants for the trainable RD29B gene; the profiles of the control ACT7 gene is shown in the panel to the right. ( f ) Rates of water loss from detached leaves of wild-type (WS) or atx1 plants during a first or fourth dehydration stresses: dark blue and red lines illustrate data for WS, first and fourth stresses, respectively; brown and light blue lines illustrate data for atx1 during the first and fourth stresses, respectively. Experiments were repeated at least twice, each with three replicates, and the representative experiment shown indicates the mean±s.e.m., n =3 replicates. Full size image An altered ability of Arabidopsis leaf cells to retain water during repetitive exposures to dehydration stress ( Fig. 1 ) as well as the increased transcriptional responses from a subset of genes ( Fig. 2 , Supplementary Fig. S1 ) illustrate the concept of a memory from an earlier stress. Our method for applying multiple dehydration stress/recovery treatments in a relatively short time, as opposed to prolonged soil–water withdrawal/recovery treatments, allowed us to observe this phenomenon and may explain why it has evaded detection in Arabidopsis so far. It is particularly relevant to point out that our experimental system is similar to the day/night oscillations in the leaf water potential that plants experience in the field during low soil water potential conditions [22] , [23] , [24] . It is tempting to suggest that under natural conditions stress memory is activated by the previous day's dehydration stress, persists through the recovery period at night (when transpiration is less and leaf water potential recovers) and then facilitates the plant's response to dehydration stress encountered during the next day, when adequate soil water is unavailable to maintain leaf water potentials at the higher transpiration rates occurring during the day. The duration of dehydration stress memory, persisting for up to 5 days in trained Arabidopsis plants recovering in watered soil ( Fig. 6 ), is sufficiently long and may be a mechanism used by plants during soil–water deficit conditions. A well-studied example of epigenetic memory in plants occurring under natural conditions is the regulation of flowering time in Arabidopsis upon vernalization, which involves repression of the homeotic FLC gene. Prolonged cold initiates pathways that are maintained for the remainder of the plant's life cycle [25] , [26] . We emphasize that the epigenetic memory at the FLC locus involves repressive polycomb group and small RNA-mediated silencing mechanisms [27] . In contrast, the vernalization-regulated transcription of the VRN1 gene is positively regulated. Its induced transcription is maintained throughout the plant development [28] , [29] but it does not show intervening periods of low transcription. The inducible transcriptional memory described here is different from the persistent expression of VRN1 , as the transcription of the trainable gene cycles in correlation with the stress or recovery conditions, indicating that memory is preserved during the low-expression recovery periods. A signature feature of the trained genes is the preservation of elevated H3K4me3 during their transcriptionally less active recovery periods. Changes in histone modifications, including H3K4me3, in response to environmental stresses have been reported for cold treatments, high salinity, hypoxia and drought-induced transcription from response genes in a variety of plant species and tissue cultures [30] , [31] , [32] . However, maintenance of these stress-induced chromatin changes after the removal of the initial signal has not been reported, except for some plant defence–response genes. H3K4me3 accumulates on the nucleosomes of defence–response genes before their induction by a pathogen attack [33] or upon chemical priming [6] , [7] . Priming leads to an increased systemic immunity response on subsequent treatments and stronger transcriptional induction of response-related genes relative to non-exposed plants [6] , [7] , [34] , [35] . Elevated H3K4me3 levels in the primed state and the subsequent stronger transcriptional response from primed defence genes resembles the transcriptional memory described here. A major difference, however, is that priming establishes H3K4me3 before activation of transcription from defence genes [6] , [7] . As such, the H3K4me3 does not occur as a mark retained from a previously active state (as with trainable genes) but, rather, appears as a 'preparatory' mark for future inductions [33] . Transcriptional memory, lasting 1–12 h and involving the H3K4me3 modification, has been reported for Saccharomyces cerevisiae genes [36] , [37] , [38] , [39] . A major distinction, however, is that the memory mechanism in yeast does not involve stalled Pol II. Stalled Ser5P Pol II during recovery from previous transcriptionally active periods is another signature feature of the Arabidopsis trained genes. This study provides the first example of a stalled Pol II at plant genes. Found at the 5′-ends of inactive metazoan developmental, or stress regulated genes, stalled (paused) Pol II has been proposed to enhance rapid transcriptional responses [40] or to allow for a synchronous induction of the same gene sets in distinct cell populations at a particular developmental stage [41] . Although the molecular mechanism is unclear, stalled Pol II is associated with the massively increased transcription during later inductions [17] . A major difference from the trainable Arabidopsis genes is that Ser5P Pol II is present at the developmental animal genes before their transcriptional activation [17] . In contrast, the Ser5P Pol II levels at the plant genes are low before induction, but remain at elevated levels across a broader region of the gene during the recovery that follows active transcription ( Fig. 4 , Supplementary Fig. S1 ). The most important remaining question is what factors cause transcriptional memory and the Ser5P and H3K4me3 association with the trainable genes. To address this question we analysed the possible involvement of ABA, a key signalling molecule in dehydration stress, of three master TFs regulated by ABA, and of the histone H3K4me3 methyltransferase, ATX1, regulating the expression of the examined genes. ABA signalling has a critical role in the dehydration stress response and regulates transcription from a large number of Arabidopsis genes [42] , including those studied here. Earlier, in genome-wide analyses, we found that the ABA-inducible genes displayed a broader H3K4me3 distribution profiles along the genes' sequences that was distinct from the typical H3K4me3 accumulation at +300 bp downstream of the transcription start sites [43] . Here we establish that this broader H3K4me3 profile is a feature of both non-trainable and trainable response genes. During each dehydration stress, endogenous ABA increased to about the same level ( Fig. 6i ), thus precluding a model wherein higher induction of ABA levels can account for the super-induction of trainable genes observed in S4 versus S1. Moreover, after 7 days of recovery in watered soil, exposure of trained plants to a dehydration stress results in a non-trained transcriptional response, despite comparable levels of ABA in plants that were dehydration stressed after recovery for 5 or 7 days ( Fig. 6a,b ). The loss of transcriptional memory by day 7 coincided with the loss of the elevated levels of Ser5P and H3K4me3 at the trainable genes. Thereby, despite the presence of high ABA levels induced by the stress, a trained transcriptional response is not displayed when the memory and signature marks are lost. We also note that during recovery, ABA levels are slightly higher than in the initial watered stage ( Fig. 6i ). Importantly, higher baseline ABA levels were present 5 days after watering when transcriptional memory was still active and were also present 7 days after watering ( Fig. 6i ) when transcriptional memory was no longer active ( Fig. 6a,b ). This result demonstrates that the higher ABA basal levels during recovery periods are not sufficient for maintaining the transcriptional memory. Therefore, we conclude that although ABA is critically required for inducing the transcriptional responses from both non-trainable and trainable genes [15] , ABA levels do not explain the super-induction of trained genes or the maintenance of transcriptional memory in the recovery state. Persistence of higher levels of key TFs after the first stress event is another potential mechanism for transcriptional memory. Our results here indicate that accumulation of active TFs is unlikely as transcript levels and transcription rates return to basal levels during the recovery (watered) phases. To assess the role of three master TFs regulated by ABA and known to induce RD29B and RAB18 during dehydration stress, we analysed dehydration stress responses in a triple mutant deficient in the AREB1, AREB2 and ABF3 genes [18] . Despite the strong reduction in transcription in RD29B and RAB18 transcript levels, the transcriptional memory response was still preserved in triple mutant plants ( Fig. 7c,d ). Thereby, although AREB1, AREB2 and ABF3 are critical for the robust response of the RD29B and RAB18 trained genes during both the initial and repetitive stress responses, they are not essential for the transcriptional memory. Finally, we emphasize that the results in the atx1 background provide independent evidence that the trainable behaviour is not directly linked to the level of transcriptional activity, as trainable genes in atx1 mutants produce reduced transcript levels and display lower levels of retained H3K4me3, while maintaining trainability ( Fig. 8 ). Thereby, the key TFs, in addition to ABA and the chromatin modifier ATX1, are not the factors causing the transcriptional memory response, although they strongly affect the magnitude of the transcriptional responses. Trainability is displayed by a distinct gene subset within the larger dehydration stress–response gene set and is associated with high levels of Ser5P Pol II and H3K4me3 during the recovery periods. The different behaviour of the trainable and non-trainable genes allows plants to modify and adjust their responses during repeated episodes of dehydration stress. Further studies would be needed to elucidate the signalling pathways and mechanisms that cause the dehydration-induced transcriptional memory in plants. Plant growth and treatments Wild-type and atx1 Arabidopsis plants were grown in potting soil in growth rooms at 22 °C with a 12-h light photoperiod and light intensity of 180 μmol m −2 s −1 . Dehydration stress was initiated by removing the plants from soil, washing any remaining soil from their roots, and then air-drying for 2 h. This exposure resulted in a decrease in fresh tissue mass to ∼ 65% of untreated (control) leaves, and is annotated as Stress1 (S1). In preliminary experiments, we have established that on reaching ∼ 65% of RWC, whole plants (or detached tissues) could recover fully on rehydration, indicating that this level of water loss is reversible and non-lethal. Additional advantage of this method is that developmental differences between the plants experiencing different numbers of stress cycles are minimized. Recovery (R1) was achieved by placing plants in humid chambers for 22 h with their roots in a few drops of water. For a subsequent stress treatment, R1 plants were gently blotted onto filter paper to remove water and air-dried for 2 h (S2) followed by a recovery (R2). The same procedures were repeated for S3, R3 and S4. Prolonged watering of 3, 5 or 7 days was accomplished by replanting the plants in soil until harvest or a terminal dehydration stress. To exclude the possibility that potential wounding of roots during extraction from soil affected the transcriptional response of the tested genes, we analysed plants removed from soil but kept in humid chambers throughout the stress–recovery cycle as controls. In the absence of dehydration stress, these control plants did not induce the dehydration stress–response genes ( Supplementary Fig. S2 ). Further, when these control plants were exposed to their first dehydration stress, they responded with induced transcript levels typical for a S1 response ( Supplementary Fig. S2 ). We concluded that potentially occurring root breakage does not have an observable effect on the dehydration stress responses we are measuring. Water loss and RWC measurements Relative water content was measured to follow the plant's water status. This value was calculated using the formula: RWC (%)=[(FW−DW)/(TW−DW)]×100% (ref. 44 ), where FW is fresh weight, DW is dry weight and TW is turgid weight. Leaves were detached from plants and immediately weighed to determine their FW. The same leaves were submerged in deionized water for 24 h, blotted dry and weighed to determine their TW. Measurements of DW were taken after the leaves were oven-dried (65 °C) in brown paper bags for 24 h. Nuclear run on assays Nuclei were isolated from the tissue ground in a mortar and pestle, following the method of Meng and Lemaux [45] , except that fresh, non-frozen tissues were used and the nuclei were purified on a 2 M sucrose pad [46] . Nuclear run on assays were performed with 0.25 mM biotin-16-UTP and 0.75 mM of ATP, CTP and GTP in the transcription reaction. The Trizol (Invitrogen, Carlsbad, CA, USA) isolated RNA was treated with DNAse I, and then purified on an RNeasy column (Qiagen, Valencia, CA, USA), and bound to streptavidin magnetic beads (Invitrogen). RNA on the washed beads was reversed transcribed with random primers, the complementary DNA eluted at 98 °C, and specific cDNA abundances were measured by quantitative PCR. The relative transcription rate of specific genes was quantitated with the 2 −ΔΔ C t calculation, according to the manufacturer's software (Bio-Rad, Hercules, CA, USA), where ΔΔ C t is the difference in the threshold cycles and the reference to UBQ10 . Primers used are shown in Supplementary Table S1 . Chromatin immunoprecipitation assay The ChIP assay was performed according to the described method [20] , [47] . The specific antibodies (1:150 dilution) used for Ser2P Pol II (ab5095, Abcam, Cambridge, MA, USA, Lot: 703307); Ser5P Pol II (ab5131, Abcam, Lot: 806890); trimethyl-H3K4 (ab1012, Abcam, Lot: GR561731-1) or H3 (ab1791, Abcam, Lot: 517990) were added for an overnight incubation at 4 °C. The antibody–protein complexes were isolated by binding to protein A or protein G beads. The washed beads were heated at 65 °C for 8 h with proteinase K to reverse the formaldehyde crosslinking and digest proteins. The sample was then extracted with phenol/chloroform and the DNA precipitated in ethanol and resuspended in water. Purified DNA was analysed by real-time PCR with gene-specific primers shown in Supplementary Table S1 . Reverse transcription and real-time PCR Total RNA isolation and reverse transcription with oligo(dT) (18418-012, Invitrogen) were performed as described previously [20] . The amounts of individual genes were measured with gene-specific primers by real-time PCR analysis with a CyclerIQ real-time PCR Instrument (Bio-Rad) and SYBR Green mixture (Bio-Rad). The relative expression or amount of specific genes was quantitated with the 2 −ΔΔ C t calculation [48] , according to the manufacturer's software (Bio-Rad), where ΔΔ C t is the difference in the threshold cycles and the reference housekeeping gene, which was ubiquitin for expression analyses or relative to input DNA for ChIP assays. The specific primers used are shown in Supplementary Table S1 . How to cite this article: Ding, Y. et al . Multiple exposures to drought 'train' transcriptional responses in Arabidopsis . Nat. Commun. 3:740 doi: 10.1038/ncomms1732 (2012).